Wnt secretion is required to maintain high levels of Wnt activity in colon cancer cells Aberrant regulation of the Wnt/β-catenin pathway has an important role during the onset and progression of colorectal cancer, with over 90% of cases of sporadic colon cancer featuring mutations in APC or β-catenin. However, it has remained a point of controversy whether these mutations are sufficient to activate the pathway or require additional upstream signals. Here we show that colorectal tumours express elevated levels of Wnt3 and Evi/Wls/GPR177. We found that in colon cancer cells, even in the presence of mutations in APC or β-catenin, downstream signalling remains responsive to Wnt ligands and receptor proximal signalling. Furthermore, we demonstrate that truncated APC proteins bind β-catenin and key components of the destruction complex. These results indicate that cells with mutations in APC or β-catenin depend on Wnt ligands and their secretion for a sufficient level of β-catenin signalling, which potentially opens new avenues for therapeutic interventions by targeting Wnt secretion via Evi/Wls. Wnt signalling pathways are highly conserved across metazoans and have important roles in many biological processes, including embryonic development, tissue homeostasis and carcinogenesis [1] . Canonical Wnt signalling through β-catenin is of particular importance for the development of colorectal cancer, with more than 80% of tumours carrying loss-of-function mutations in adenomatous polyposis coli (APC) and about 5% carrying activating mutations in β-catenin [2] , [3] . In the normal intestinal epithelium, Wnt signalling regulates the proliferation and differentiation of intestinal stem and progenitor cells. Mutations in APC and β-catenin are among the earliest events of colon cancer development and lead to hyperplasia in the intestinal crypts [4] , [5] . Recent studies have shown that Wnt signalling activity is also required in colon cancer cells during tumour progression and metastasis [6] . The secretion of Wnt proteins requires Evenness interrupted/Wntless/G protein-coupled receptor 177 (Evi/Wls/GPR177) [7] , [8] , [9] , [10] , [11] . This multipass transmembrane protein acts as a cargo receptor for Wnt proteins, shuttling them from the Golgi to the plasma membrane where they act in an autocrine or paracrine manner to activate Wnt signalling pathways. Upon binding to receptors of the Frizzled family and their coreceptors, Wnt proteins activate different downstream signalling pathways. In the so-called canonical pathway, signals are transmitted through Dishevelled (Dvl) adaptor proteins, leading to the stabilization of cytosolic β-catenin and its translocation to the nucleus. In the absence of Wnt signalling, β-catenin degradation is initiated by the ‘destruction complex’, which comprises, among other proteins, APC, GSK3β and Axin1. APC acts as a scaffold, binding β-catenin and recruiting CK1α and GSK3β to phosphorylate β-catenin. This event marks β-catenin for ubiquitination by the SKP1–Cullin-1–F-box (SCF βKP1- ) E3 ubiquitin ligase complex and subsequently triggers its proteasomal degradation [12] . When β-catenin translocates to the nucleus as a consequence of Wnt signalling, it acts as a cofactor for transcription factors of the T-cell factor (TCF) family, leading to the transcription of Wnt/β-catenin target genes such as AXIN2 , SMAD7 , CCND1 / CyclinD and MYC . Given that mutations in APC and β-catenin are thought to lead to a constitutively active Wnt pathway that renders cells insensitive to upstream regulation, many drug development efforts for colon cancer have focused on downstream targets [2] , [13] . However, other experimental data challenge the assumption that mutant APC alone is sufficient to sustain Wnt pathway activity. For example, secreted Wnt antagonists such as the secreted Frizzled-related proteins (SFRPs) have been found to attenuate Wnt/β-catenin signalling in colorectal cancer cell lines carrying APC mutations [14] , [15] ; this observation has also been explained by proposing novel, Wnt/β-catenin-independent functions for these factors [16] , [17] . Other studies have shown that β-catenin expression patterns across a colon tumour are heterogeneous, suggesting that the Wnt pathway activity across a tumour can be variable irrespective of the homogeneous distribution of the activated β-catenin mutant protein throughout that tumour [18] , [19] , [20] , [21] . These observations highlight the need to dissect the mechanisms that underlie the effects of APC and β-catenin mutations on the Wnt/β-catenin signalling cascade. Here we show that the levels of both Wnt3 and Evi/Wls are frequently higher in adenomas and differentiated carcinomas than in normal colon epithelium. We also demonstrate that interfering with the secretion of Wnt proteins in colon cancer cell lines that harbour APC or β-catenin mutations impairs the ability of the cells to proliferate and to form colonies in vitro and tumours in vivo . We provide evidence that autocrine Wnt secretion via Evi/Wls is required for maintaining the Wnt activity in cell lines and tumour-initiating cells (TICs). Taken together, these results support a model, wherein colon cancer cells acquire the ability to secrete canonical Wnt proteins continuously, and require such autocrine secretion for survival. Evi/Wls and Wnt3 are highly expressed in colon carcinomas In the normal mouse small intestinal epithelium, Wnt3 is highly expressed in Paneth cells where it has a crucial role in maintaining LGR5 + intestinal stem cells at the bottom of the crypt [22] , [23] . Here we asked whether a similar expression pattern of Wnt3 and its cargo receptor Evi/Wls can be detected in human colon tissue. To this end, we stained normal human colon and matched carcinoma tissue sections (from the same patient) for Wnt3 and Evi/Wls protein, using Keratin20 and Eph receptor B2 as markers of cell differentiation ( Fig. 1a,b and Supplementary Fig. S1b ) [24] . We found that Wnt3 and Evi/Wls proteins were low or were not detectable in enterocytes and goblet cells, whereas their expression was more prominent in the underlying lamina muscularis mucosae ( Fig. 1a ). In addition, high Wnt3 expression was observed in scattered cells, which showed characteristics of endocrine and Paneth-like [25] cells localized at the bottom of the crypt, with eosinophilic granula in the cytoplasm and the basal nuclei. These results suggest that an important source of Wnt proteins in the human colon is located at the bottom end of the crypts. 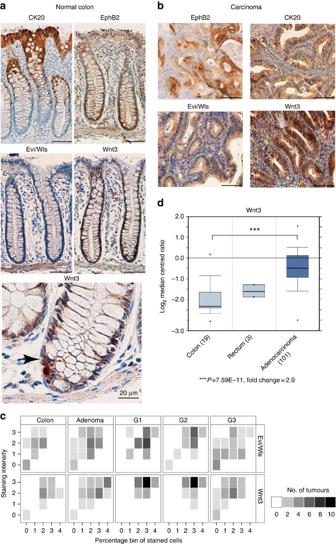Figure 1: Evi/Wls is highly expressed in colon tumours. (a,b) Immunohistochemical staining of normal or carcinoma tissue sections from colon, using the indicated antibodies. Images are representative of five cases. (a) In normal tissue, Evi/Wls expression is mostly undetectable, whereas Wnt3 is weakly expressed in most epithelial cells but more highly expressed in the Paneth-like/endocrine cells, which have a granular appearance (arrow). Keratin20 staining marks the top of the intestinal crypts and Eph receptor B2 staining the bottom. (b) In matched colon carcinomas, Evi/Wls and Wnt3 are highly expressed. (a,b) Scale bars, 60 μm, Wnt3 (enlarged) 20 μm. (c) Evi/Wls and Wnt3 are overexpressed in colon cancer. Results of immunostainings for Evi/Wls and Wnt3 on a colon cancer tissue array. Scores provided independently by three different investigators are shown as average. Staining intensity: 0=no staining, 1=weak staining, 2=moderate staining, 3=strong staining; percentage bin of cells: 0=<10%, 1=10–25%, 2=25–50%, 3=50–75%, 4=>75%). Grey scale represents the number of tumours. (d) Wnt3 is overexpressed in adenocarcinomas. Microarray-based expression data (Oncomine database, TCGA data set) were analysed for the expression of Wnt3 in normal colon(19)/rectum(3) versus adenocarcinomas (101). Preprocessed data from the array is log2-transformed and median-centred. The box plots show medians as line within the box, 25th and 75th percentiles as sides of the box, 10th and 90th percentiles as error bars, and outliers as circles. Significance of the differences in expression was calculated using the Student’st-test. The specificity of the Wnt3 antibody was tested by knockdown experiments (Supplementary Fig. S1a). Evi/Wls antibody is described in Augustinet al.10 Figure 1: Evi/Wls is highly expressed in colon tumours. ( a , b ) Immunohistochemical staining of normal or carcinoma tissue sections from colon, using the indicated antibodies. Images are representative of five cases. ( a ) In normal tissue, Evi/Wls expression is mostly undetectable, whereas Wnt3 is weakly expressed in most epithelial cells but more highly expressed in the Paneth-like/endocrine cells, which have a granular appearance (arrow). Keratin20 staining marks the top of the intestinal crypts and Eph receptor B2 staining the bottom. ( b ) In matched colon carcinomas, Evi/Wls and Wnt3 are highly expressed. ( a , b ) Scale bars, 60 μm, Wnt3 (enlarged) 20 μm. ( c ) Evi/Wls and Wnt3 are overexpressed in colon cancer. Results of immunostainings for Evi/Wls and Wnt3 on a colon cancer tissue array. Scores provided independently by three different investigators are shown as average. Staining intensity: 0=no staining, 1=weak staining, 2=moderate staining, 3=strong staining; percentage bin of cells: 0=<10%, 1=10–25%, 2=25–50%, 3=50–75%, 4=>75%). Grey scale represents the number of tumours. ( d ) Wnt3 is overexpressed in adenocarcinomas. Microarray-based expression data (Oncomine database, TCGA data set) were analysed for the expression of Wnt3 in normal colon(19)/rectum(3) versus adenocarcinomas (101). Preprocessed data from the array is log 2 -transformed and median-centred. The box plots show medians as line within the box, 25th and 75th percentiles as sides of the box, 10th and 90th percentiles as error bars, and outliers as circles. Significance of the differences in expression was calculated using the Student’s t -test. The specificity of the Wnt3 antibody was tested by knockdown experiments ( Supplementary Fig. S1a ). Evi/Wls antibody is described in Augustin et al. [10] Full size image Surprisingly, in carcinoma sections from the same patients, Evi/Wls and Wnt3 staining was stronger and detectable throughout the epithelium ( Fig. 1b ). To confirm these data, we also stained tumour tissue arrays for Evi/Wls and Wnt3 ( Fig. 1c ; representative immunohistochemical stainings are shown in Supplementary Fig. S1b ). Wnt3 and Evi/Wls expression in the epithelial cells of normal colon tissue (colon) was generally weaker compared with tumuor tissues. However, it was elevated in adenomas and showed strong expression in well- (G1) and moderately (G2) differentiated (adeno-) carcinomas, whereas poorly (G3) differentiated tumours showed heterogeneous Evi/Wls expression ( Fig. 1c ). Our expression data are also consistent with the TCGA messenger RNA expression data set (Oncomine, www.oncomine.org , TCGA) [3] , which shows that the Wnt3, Wnt1 and Wnt3a mRNAs ( Fig. 1d and Supplementary Fig. S1c ) are more highly expressed in colorectal adenocarcinomas than in normal colon/rectum. Next, we tested whether overexpressing the cargo receptor Evi/Wls in colon cancer cells leads to an increase in Wnt signalling activity, as previously shown in embryonic stem (ES) cells [10] . As illustrated in Supplementary Fig. S1d , the overexpression of Evi/Wls in the colon cancer cell line HCT116 led to a twofold increase in Wnt reporter activity, indicating that the increased secretion of Wnt proteins can upregulate canonical signalling. Taken together, our data provide evidence that Wnt secretion could have a functional role in colorectal carcinomas, and that colorectal carcinoma cells have acquired the ability to secrete Wnt ligands in an autocrine manner. Evi is required for high levels of Wnt pathway activation To investigate the requirements for Evi/Wls expression in colon cancer cells that harbour mutations in APC or β-catenin, we chose two colon cancer cell lines: DLD1 (APC mutation; truncated protein) and HCT116 (β-catenin mutation, loss of phosphorylation site S45). Short hairpin RNA (shRNA)-mediated silencing of the Evi/Wls significantly reduced lymphoid enhancer factor (LEF)/Wnt-reporter [26] induction to levels comparable to those achieved by Bcl9 knockdown, an essential transcriptional cofactor for the expression of Wnt/β-catenin target genes ( Fig. 2a and Supplementary Fig. S2a ). This effect was rescued by adding recombinant Wnt3a ( Supplementary Fig. S2b ). Furthermore, knockdown of Evi/Wls with a doxycycline (dox)-inducible shmirRNA led to downregulation of the canonical Wnt target gene AXIN2 in both DLD1 and HCT116 cells ( Fig. 2b ), an effect that was likewise rescued by applying recombinant Wnt3a ( Supplementary Fig. S2c,d ). 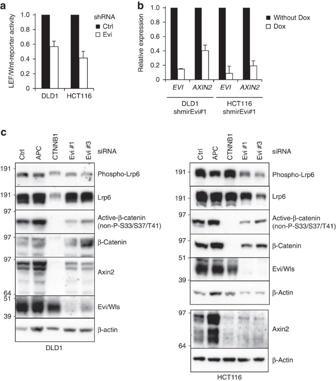Figure 2: Evi/Wls is required to maintain canonical Wnt signalling in colon cancer cell lines. (a) Evi/Wls depletion reduces canonical Wnt signalling. DLD1 and HCT116 TCF4/Wnt reporter-colon cancer cells were transduced with lentivirus introducing a control or Evi shRNA construct. Luciferase assay was normalized to viability assessed in parallel using the CellTiterGlo assay. Results of three (for DLD1) and five (for HCT116) independent experiments are shown as mean±s.e.m. (b) Silencing of Evi/Wls regulates the Wnt target gene expression. DLD1 and HCT116 cells were transduced with a dox-inducible shmirEvi#1 construct and treated with or without dox. After 96 h, the cells were analysed for the expression ofAXIN2andEVI/WLSmRNAs by quantitative PCR. Results of four independent experiments are shown as mean±s.e.m. (c) Silencing of Evi/Wls reduces the level of active β-catenin in DLD1 and HCT116 cells, which express mutated APC or β-catenin, respectively. DLD1 cells were transfected with the indicated siRNAs for 120 h, and HCT116 cells were transfected for 72 h. Subsequently, the cells were lysed and western blotting was performed with the indicated antibodies. β-Actin served as the loading control. The reduction of total Lrp6 in β-catenin knockdown cells, which is consistently observed in DLD1 cells, may be a consequence of reduced β-catenin levels at the adherent junctions59. Figure 2: Evi/Wls is required to maintain canonical Wnt signalling in colon cancer cell lines. ( a ) Evi/Wls depletion reduces canonical Wnt signalling. DLD1 and HCT116 TCF4/Wnt reporter-colon cancer cells were transduced with lentivirus introducing a control or Evi shRNA construct. Luciferase assay was normalized to viability assessed in parallel using the CellTiterGlo assay. Results of three (for DLD1) and five (for HCT116) independent experiments are shown as mean±s.e.m. ( b ) Silencing of Evi/Wls regulates the Wnt target gene expression. DLD1 and HCT116 cells were transduced with a dox-inducible shmirEvi#1 construct and treated with or without dox. After 96 h, the cells were analysed for the expression of AXIN2 and EVI/WLS mRNAs by quantitative PCR. Results of four independent experiments are shown as mean±s.e.m. ( c ) Silencing of Evi/Wls reduces the level of active β-catenin in DLD1 and HCT116 cells, which express mutated APC or β-catenin, respectively. DLD1 cells were transfected with the indicated siRNAs for 120 h, and HCT116 cells were transfected for 72 h. Subsequently, the cells were lysed and western blotting was performed with the indicated antibodies. β-Actin served as the loading control. The reduction of total Lrp6 in β-catenin knockdown cells, which is consistently observed in DLD1 cells, may be a consequence of reduced β-catenin levels at the adherent junctions [59] . Full size image RNA interference (RNAi)-mediated downregulation of Evi/Wls reduced the phosphorylation of Lrp6 on Ser1490 in both DLD1 and HCT116 cells, confirming that pathway activity was reduced at the receptor level ( Fig. 2c ) [27] , [28] . Evi/Wls depletion in these cell lines also reduced the levels of active β-catenin (non-phosphorylated-S33/S37/T41) and of Axin2 ( Fig. 2c ). To confirm the specificity of knockdown, we rescued Wnt pathway activation in HEK293T cells after knockdown of Evi/Wls, using modified Evi/Wls expression constructs [29] not targeted by the short interfering RNAs (siRNAs; Supplementary Fig. S3a ). These findings suggest that Evi/Wls activity contributes to the activation of canonical Wnt signalling in the presence of an APC or β-catenin mutation. Next, we tested whether blocking Wnt secretion using IWP12, an inhibitor of the porcupine protein, the Wnt acyl-transferase [30] , [31] , interferes with Wnt activity in HCT116 cells. The results presented in Supplementary Fig. S3b were similar to those obtained for Evi/Wls silencing, supporting a model wherein Wnt secretion is required for the activity of the canonical Wnt pathway. Recently, it has been shown that R-spondins bind to Lgr5 to activate Wnt signalling [32] , [33] , [34] . Thus, we tested whether the effect of Evi/Wls silencing can be rescued by adding recombinant R-spondin1. As shown in Supplementary Fig. S3c–e , R-spondin1 could not rescue Wnt signalling in colon cancer cells when Evi/Wls was depleted, in contrast to control experiments. In summary, these results indicate that even in the presence of the APC or β-catenin mutations, canonical Wnt signalling in colon cancer cells depends on Wnt secretion. Depletion of Evi/Wls leads to an almost complete loss of canonical Wnt pathway activity, which cannot be rescued by the addition of R-spondin. Mutated APC and upstream regulation of Wnt signalling Next, we investigated whether the presence of Wnts is required for canonical signalling in colon cancer cell lines with mutant APC. RNAseq data from seven colon cancer cell lines indicated that several canonical Wnt ligands are expressed in each cell line, the most prominent among these being Wnt3 and Wnt10b ( Supplementary Fig. S4a ). To test whether these ligands are secreted and functional, we cocultured SW480 and DLD1 cells with a MDA-MB231 or HEK293T reporter cell line. We found that both colon cancer cell lines induced canonical Wnt signalling in a cell-number-dependent manner ( Fig. 3a and Supplementary Fig. S4b,c ), producing a range of reporter activity similar to that observed when recombinant Wnt3a was applied ( Supplementary Fig. S4b ). To exclude the possibility of confounding effects from increased reporter cell proliferation, we assessed the activity of a TCF/LEF–GFP reporter at the single-cell level by fluorescence-activated cell sorting. Consistent with our results from the luciferase assays, coculturing the reporter cell line with SW480 cells enhanced TCF/LEF–GFP fluorescence in reporter cells in a dose-dependent manner ( Supplementary Fig. S5a ). These experiments indicated that colon cancer cells secrete functional Wnt proteins. 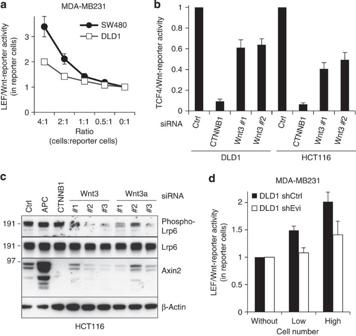Figure 3: Wnt secretion is required to maintain canonical Wnt signalling in colon cancer cell lines. (a) DLD1 and SW480 colon cancer cells activate the Wnt pathway in cocultured MDA-MB231 reporter cells. DLD1 or SW480 cells were cocultured with MDA-MB231 reporter cells stably transduced with a TCF/LEF reporter (1,500 cells) at the indicated ratio for 48 h. Next, cells were lysed and luciferase activity was measured. (b) Silencing of Wnt3 in DLD1 and HCT116 cells stably transfected with a TCF4/Wnt reporter reduces canonical Wnt signalling activity. Both cell lines were transfected with the indicated siRNAs. HCT116 cells were incubated for 72 h and DLD1 cells for 96 h before read-out. Luciferase levels were normalized to cell survival assessed by a CellTiterGlo assay performed in parallel. (c) Silencing of Wnt3a or Wnt3 reduces Axin2 protein expression. HCT116 cells were transfected with the indicated siRNAs for 72 h. Cell lysates were used for western blotting with indicated antibodies. β-Actin served as the loading control. (d) Evi/Wls knockdown in DLD1 cells reduces the induction of TCF/LEF reporter activity in coseeded MDA-MB231 reporter cells. Coculture of cells was conducted as described ina. Half times more DLD shEvi cells than shCtrl cells were seeded to compensate for reduced viability. (a,b,d) Data from three independent experiments are presented as mean±s.e.m. Figure 3: Wnt secretion is required to maintain canonical Wnt signalling in colon cancer cell lines. ( a ) DLD1 and SW480 colon cancer cells activate the Wnt pathway in cocultured MDA-MB231 reporter cells. DLD1 or SW480 cells were cocultured with MDA-MB231 reporter cells stably transduced with a TCF/LEF reporter (1,500 cells) at the indicated ratio for 48 h. Next, cells were lysed and luciferase activity was measured. ( b ) Silencing of Wnt3 in DLD1 and HCT116 cells stably transfected with a TCF4/Wnt reporter reduces canonical Wnt signalling activity. Both cell lines were transfected with the indicated siRNAs. HCT116 cells were incubated for 72 h and DLD1 cells for 96 h before read-out. Luciferase levels were normalized to cell survival assessed by a CellTiterGlo assay performed in parallel. ( c ) Silencing of Wnt3a or Wnt3 reduces Axin2 protein expression. HCT116 cells were transfected with the indicated siRNAs for 72 h. Cell lysates were used for western blotting with indicated antibodies. β-Actin served as the loading control. ( d ) Evi/Wls knockdown in DLD1 cells reduces the induction of TCF/LEF reporter activity in coseeded MDA-MB231 reporter cells. Coculture of cells was conducted as described in a . Half times more DLD shEvi cells than shCtrl cells were seeded to compensate for reduced viability. ( a , b , d ) Data from three independent experiments are presented as mean±s.e.m. Full size image Next, we investigated whether the Evi/Wls phenotype is equivalent to that resulting from the loss of canonical Wnts. Depleting HCT116 cells of Wnt3 and Wnt3a, and DLD1 cells of Wnt3 ( Fig. 3b ), strongly reduced the reporter activity. Silencing of Wnt3a was rescued by adding recombinant Wnt3a ( Supplementary Fig. S5b ). Combined knockdown of both Wnt3 and Wnt3a led to a further reduction of Wnt signalling ( Supplementary Fig. S5c ). We also observed reduced expression of the Wnt target genes AXIN2 and SMAD7 ( Supplementary Fig. S5d ), a reduction of Lrp6 phosphorylation (Ser1490) and a decrease in Axin2 protein levels ( Fig. 3c ) after RNAi-mediated silencing of Wnt3 or Wnt3a. As expected, the ability of the Wnt ligands to activate signalling was dependent on the presence of Evi/Wls in the secreting cells ( Fig. 3d ). Consistent with these findings, silencing of Lrp6, Dvl1 and Dvl3 led to a decrease in TCF4/Wnt-reporter activity, despite the presence of APC and β-catenin mutations ( Fig. 4a ), and silencing of Dvl1 and Dvl3 led to downregulation of AXIN2 mRNA ( Fig. 4b ). 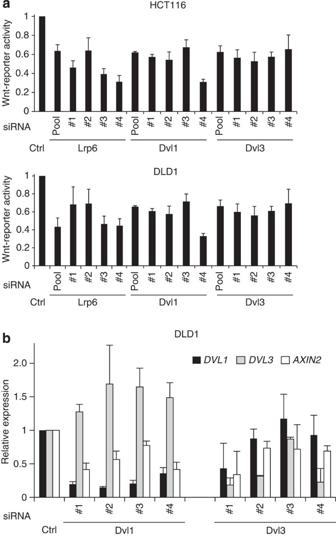Figure 4: Wnt pathway components at the receptor level are required for canonical activation in colon cancer cells. (a) Knockdown of Lrp6, Dvl1 or Dvl3 reduces Wnt reporter activity in HCT116 and DLD1 cells. Cells stably transfected with a TCF4/Wnt reporter were reverse transfected with the indicated siRNAs and assessed for luciferase activity 72 h later. (b) Silencing of Dvl1 and Dvl3 reduces Wnt target gene expression in DLD1 cells. DLD1 cells were reverse transfected with the indicated siRNA and assessed for the expression of the Wnt target gene (AXIN2), as well asDVL1andDVL3, by quantitative PCR 72 h later. (a,b) Data from four to five independent experiments are shown as mean±s.e.m. Figure 4: Wnt pathway components at the receptor level are required for canonical activation in colon cancer cells. ( a ) Knockdown of Lrp6, Dvl1 or Dvl3 reduces Wnt reporter activity in HCT116 and DLD1 cells. Cells stably transfected with a TCF4/Wnt reporter were reverse transfected with the indicated siRNAs and assessed for luciferase activity 72 h later. ( b ) Silencing of Dvl1 and Dvl3 reduces Wnt target gene expression in DLD1 cells. DLD1 cells were reverse transfected with the indicated siRNA and assessed for the expression of the Wnt target gene ( AXIN2 ), as well as DVL1 and DVL3 , by quantitative PCR 72 h later. ( a , b ) Data from four to five independent experiments are shown as mean±s.e.m. Full size image In summary, colon cancer cell lines express canonical Wnt ligands, whose Evi/Wls-dependent secretion is regulating canonical Wnt signalling, regardless of the presence of mutated APC or β-catenin. Truncated APC can regulate canonical Wnt pathway Eighty per cent of colon cancers have biallelic APC mutations [35] , often with complete lack of expression from one allele and expression of a truncated from the other. Previous studies have indicated that depletion of APC in colon cancer cells can activate canonical Wnt signalling [36] , [37] , [38] , [39] . To test whether truncated APC alleles have residual ability to regulate downstream Wnt signalling components and whether such activity can be reduced further, we assessed the effect of RNAi-mediated APC silencing on TCF/LEF and TCF4/Wnt reporter levels in DLD1, HT29 and HCT116 cells ( Supplementary Fig. S6a ). In each of these cell lines, reducing APC expression induced reporter expression. We observed a particularly strong effect in HT29 cells, in which the truncated APC protein is longer than that in DLD1 cells ( Supplementary Fig. S6a ). In general, induction of AXIN2 mRNA appeared to correlate with the length of the truncated APC proteins ( Fig. 5a ), although we cannot completely exclude the possibility that variability in RNAi efficiency affected the results obtained for different cell lines ( Supplementary Fig. S5b ). APC silencing in DLD1 cells with different distinct APC siRNAs led to reproducible upregulation of AXIN2 ( Supplementary Fig. S6c ). These results are consistent with previous studies showing that truncated APC proteins remain capable of modulating the Wnt pathway signalling. 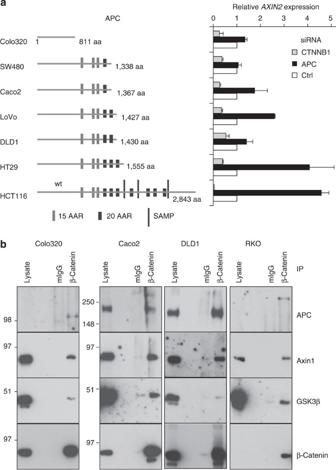Figure 5: Truncated APC in colon cancer cells is functional. (a) Silencing of mutated APC in colon cancer cells increasesAXIN2expression. Schematic representation of the APC mutant proteins that are present in various colon cancer cell lines. All mutated APC proteins lack the SAMP (serine alanine methionine proline) repeats attributed to Axin binding. HT29 cells express the longest form of APC (1,555 aa); it retains all 15 AARs, as well as three of the seven 20 AARs, all of which are responsible for β-catenin binding/degradation. The indicated colon cancer cells were transfected with CTNNB1 or APC siRNAs for 72 h. Relative expression of the indicated mRNAs was determined by quantitative PCR. Data from three to four independent experiments are shown as mean±s.e.m. (b) β-Catenin binds to the main components of the destruction complex in colon cancer cells. The indicated cell lines were subjected to immunoprecipitation with anti-β-catenin antibody. Regardless of the extent of APC truncation, β-catenin co-immunoprecipitated APC, Axin1 and GSK3β. Western blottings are shown as representative of three independent experiments using the indicated antibodies. Figure 5: Truncated APC in colon cancer cells is functional. ( a ) Silencing of mutated APC in colon cancer cells increases AXIN2 expression. Schematic representation of the APC mutant proteins that are present in various colon cancer cell lines. All mutated APC proteins lack the SAMP (serine alanine methionine proline) repeats attributed to Axin binding. HT29 cells express the longest form of APC (1,555 aa); it retains all 15 AARs, as well as three of the seven 20 AARs, all of which are responsible for β-catenin binding/degradation. The indicated colon cancer cells were transfected with CTNNB1 or APC siRNAs for 72 h. Relative expression of the indicated mRNAs was determined by quantitative PCR. Data from three to four independent experiments are shown as mean±s.e.m. ( b ) β-Catenin binds to the main components of the destruction complex in colon cancer cells. The indicated cell lines were subjected to immunoprecipitation with anti-β-catenin antibody. Regardless of the extent of APC truncation, β-catenin co-immunoprecipitated APC, Axin1 and GSK3β. Western blottings are shown as representative of three independent experiments using the indicated antibodies. Full size image Truncated APC retains functions in regulating Wnt signalling Our experiments indicated that colon cancer cell lines require canonical Wnt ligands for full pathway activation and cell survival, regardless of the presence of mutations in APC or β-catenin. We hypothesized that the mutant proteins might retain partial function, shifting the balance between activators and inhibitors of the Wnt/β-catenin pathway, rendering it more sensitive to changes in signal flow from upstream components. Previous work using overexpression constructs of APC fragments showed that it can retain β-catenin binding ability and reduce signalling activity [40] , [41] , [42] . Su et al. [43] also proposed that mutated APC has impaired function in transferring phosphorylated β-catenin for ubiquitylation. We therefore examined the biochemical effects of clinically found mutant forms of endogenous APC on destruction complex formation and Wnt/β-catenin pathway activity. As knockdown of truncated APC (1,360–1,560 aa) led to an increased expression of the Wnt target gene AXIN2 ( Fig. 5a ) [36] , [37] , [39] , we hypothesized that this protein may retain its ability to act as a scaffold for components of the destruction complex. We tested this by immunoprecipitating the destruction complex from Colo320, Caco2, DLD1 and RKO cells (truncations of 811, 1,367 and 1,430 aa, and full-length APC, respectively). As shown in Fig. 5b , endogenous APC, Axin1 and GSK3β co-immunoprecipitated with β-catenin in all cases, indicating that these truncated APC proteins retain the ability to bind β-catenin. Next, we evaluated whether the truncated APC proteins supported the formation of destruction complex and induced phosphorylation of β-catenin. We co-immunoprecipitated endogenous APC, Axin1 and GSK3β from DLD1 and SW480 cells. We detected β-catenin phosphorylation at sites S33 and S37 (as also shown in refs 43 , 44 ), as well as the presence of the major components of the destruction complex ( Fig. 6a and Supplementary Fig. S7a ), indicating that truncated APC proteins are partly functional. Thus, loss of β-catenin-binding sites in colon cancer cells, such as DLD1 and SW480, leads to a reduction in APC levels rather than its complete inactivation. 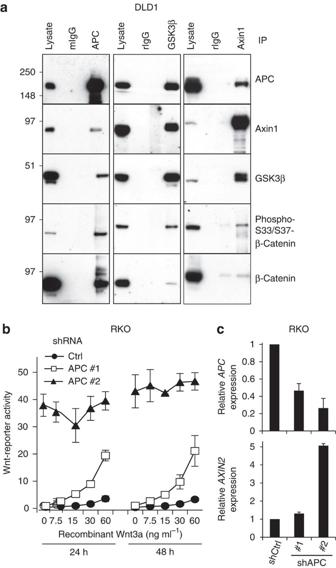Figure 6: Cells expressing truncated APC can form a functional destruction complex. (a) β-Catenin bound to the main components of the destruction complex in DLD1 cells is phosphorylated. DLD1 cells were subjected to immunoprecipitation with anti-APC, -GSK3β or -Axin1 antibody. Western blottings are representative of three independent experiments. (b,c) A moderate decrease in APC level is not sufficient to induce Wnt signalling, but sensitizes cells to Wnt3a. RKO colon cancer cells that express wild-type APC and are stably transfected with a TCF4/Wnt reporter were transduced with the indicated shRNA constructs. (b) Luciferase activity was measured in RKO TCF4/Wnt cells treated with the indicated amounts of recombinant Wnt3a protein for 24 or 48 h. (c) Relative expression ofAPCandAXIN2was measured by quantitative PCR. (b,c) Results of six (b) and three (c) independent experiments are shown as mean±s.e.m. Figure 6: Cells expressing truncated APC can form a functional destruction complex. ( a ) β-Catenin bound to the main components of the destruction complex in DLD1 cells is phosphorylated. DLD1 cells were subjected to immunoprecipitation with anti-APC, -GSK3β or -Axin1 antibody. Western blottings are representative of three independent experiments. ( b , c ) A moderate decrease in APC level is not sufficient to induce Wnt signalling, but sensitizes cells to Wnt3a. RKO colon cancer cells that express wild-type APC and are stably transfected with a TCF4/Wnt reporter were transduced with the indicated shRNA constructs. ( b ) Luciferase activity was measured in RKO TCF4/Wnt cells treated with the indicated amounts of recombinant Wnt3a protein for 24 or 48 h. ( c ) Relative expression of APC and AXIN2 was measured by quantitative PCR. ( b , c ) Results of six ( b ) and three ( c ) independent experiments are shown as mean±s.e.m. Full size image We also investigated whether a reduction in APC functionality, although insufficient to activate the pathway on its own, sensitizes cells to the Wnt ligands. We used RKO that expresses wild-type APC and shows only basal Wnt pathway activity as a model system. To assess the effects of a partial reduction of APC levels, we stably transduced RKO TCF4/Wnt-reporter cells with shRNA constructs that target APC at different efficiencies of knockdown, as assessed by their effects on expression of the AXIN2 mRNA ( Fig. 6b,c ). We found that efficient reduction of APC expression (85% reduction, shAPC#2) induced strong reporter activity, even in the absence of the Wnt3a ligand. In contrast, moderate downregulation of APC expression (50% reduction, shAPC#1) did not induce the reporter by itself, but resulted in a stronger response when combined with exposure to Wnt3a ligand ( Fig. 6b ). We further tested the effects of APC levels in HEK293T cells that had been transfected with various siAPCs and treated with Wnt3a. Although partial silencing of APC (using either siAPC#1 or siAPC pool) did not induce TCF4/Wnt-reporter activity on its own, we observed a stronger induction when combined with Wnt3a treatment ( Supplementary Fig. S7b,c ). Together, these findings indicate that colon cancer cells expressing truncated APC can assemble a partially functional destruction complex. We conclude that truncated APC does not lead to full pathway activation, but can instead sensitize cells to upstream signals. Evi is required for the proliferation of colon cancer cells To evaluate whether Wnt secretion is required for the proliferation of colon cancer cells, we stably transduced colon cancer cell lines with lentiviral shRNA constructs targeting the Wnt cargo receptor Evi/Wls. Knockdown of Evi/Wls reduced the viability of HCT116 cells compared with cells treated with control shRNAs and the cells accumulated in G2 phase, similar to cells deficient for β-catenin ( Supplementary Figs S8 and S9a ). Comparable viability effects were observed in cells expressing truncated forms of APC ( Supplementary Fig. S9b,c ). To study the effect of Evi/Wls downregulation on long-term cell survival, we performed clonogenicity assays in HCT116, DLD1 and SW480 cells. As shown in Fig. 7a , Evi/Wls knockdown decreased colony formation relative to that measured in controls. 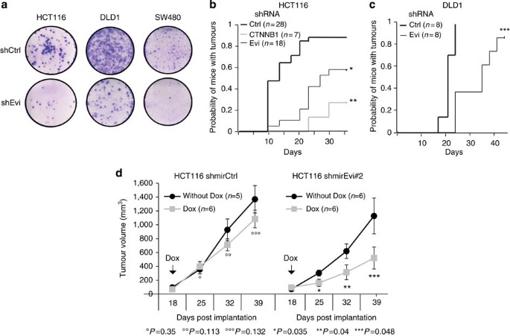Figure 7: Evi/Wls is required for the survival of colon cancer cellsin vitroandin vivo. (a) Stable Evi/Wls knockdown reduces the clonogenic capacity of colon cancer cells. HCT116, DLD1 and SW480 cells stably transduced with a control (Ctrl) or an Evi shRNA were seeded in six-well plates at 1,000 cells per well, and were stained with crystal violet 14–20 days later. Wells are representative of three independent experiments for each cell line. (b,c) Evi/Wls is required for the formation of primary colon carcinomas in a xenograft mouse model. HCT116 or DLD1 cells were transduced as described ina, were injected subcutaneously (s.c.) into NOD/SCID mice (3 × 105per mouse) and tumour appearance was monitored over time. Kaplan–Meier plots show the probability of tumour appearance over time. (b) Results from two blinded, independent experiments are shown. CTNNB1 silencing was performed just in one of these experiments. (c) Results from one blinded experiment are shown.n, number of mice per group. *P=0.000201, **P=0.0000354 and ***P=0.0015.P-values were determined by log-rank test. (d) Evi/Wls downregulation reduces tumour volumein vivo. HCT116 cells were transduced as described inaand were injected s.c. (2 × 106per mouse) into opposite flanks of the same NOD/SCID mice. Eighteen days later, when tumour volumes had reached about 120 mm3, the mice were randomly separated into two groups: one was treated with dox (added to the drinking water) and the other was not. Tumour volume was measured on a weekly basis and the significance for each time point was calculated using the Student’st-test. The experiment was terminated when tumours in the control group reached about 1,200 mm3. Results are presented as mean tumour volume±s.e.m. Figure 7: Evi/Wls is required for the survival of colon cancer cells in vitro and in vivo . ( a ) Stable Evi/Wls knockdown reduces the clonogenic capacity of colon cancer cells. HCT116, DLD1 and SW480 cells stably transduced with a control (Ctrl) or an Evi shRNA were seeded in six-well plates at 1,000 cells per well, and were stained with crystal violet 14–20 days later. Wells are representative of three independent experiments for each cell line. ( b , c ) Evi/Wls is required for the formation of primary colon carcinomas in a xenograft mouse model. HCT116 or DLD1 cells were transduced as described in a , were injected subcutaneously (s.c.) into NOD/SCID mice (3 × 10 5 per mouse) and tumour appearance was monitored over time. Kaplan–Meier plots show the probability of tumour appearance over time. ( b ) Results from two blinded, independent experiments are shown. CTNNB1 silencing was performed just in one of these experiments. ( c ) Results from one blinded experiment are shown. n , number of mice per group. * P =0.000201, ** P =0.0000354 and *** P =0.0015. P -values were determined by log-rank test. ( d ) Evi/Wls downregulation reduces tumour volume in vivo . HCT116 cells were transduced as described in a and were injected s.c. (2 × 10 6 per mouse) into opposite flanks of the same NOD/SCID mice. Eighteen days later, when tumour volumes had reached about 120 mm 3 , the mice were randomly separated into two groups: one was treated with dox (added to the drinking water) and the other was not. Tumour volume was measured on a weekly basis and the significance for each time point was calculated using the Student’s t -test. The experiment was terminated when tumours in the control group reached about 1,200 mm 3 . Results are presented as mean tumour volume±s.e.m. Full size image To assess the requirement of Evi/Wls in the survival of colon cancer cells in vivo , we injected shRNA-transduced HCT116 or DLD1 cells ( Fig. 7b,c ) subcutaneously into NOD/SCID (non-obese diabetic/severe-combined immunodeficiency) mice. Expression of the Evi shRNA delayed or abrogated tumour formation during the observation period ( P =0.000201, log-rank test), an effect that was confirmed with dox-inducible shmirRNA constructs (shmirEvi#1 and #2; Fig. 7d and Supplementary Fig. S9d ). These results demonstrate that silencing of the Wnt cargo receptor Evi/Wls reduced both the initial engraftment of the tumour and subsequent tumour growth. Evi is important for the survival of colon cancer stem cells Vermeulen et al. [21] showed that colon cancer stem cells are characterized by high Wnt activity, which is essential for stemness capacity of these cells. We hypothesized that Wnt signalling in these cells might be dependent on canonical Wnts and Evi/Wls expression in an autocrine or a paracrine manner, even in the presence of APC mutation. To investigate the role of Wnt secretion in TICs, we enriched these cells from primary human colorectal cancer tissue or derived metastases from three patients (P1–3) in serum-free medium in the presence of cytokines. Under these conditions, floating tumour spheroids are formed, which are enriched for self-renewing TICs and depleted of non-neoplastic cells [45] . P1 and P3 TICs harbour a truncated APC, whereas in P2 cells no truncations of APC was detected ( Fig. 8a ). We confirmed that the three TICs expressed Evi/Wls and Wnt3 on an mRNA level. 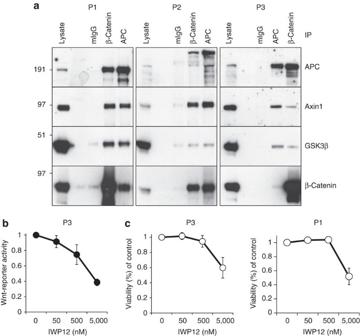Figure 8: Wnt secretion is important for the survival of colon TICs. (a) Destruction complex is functional in primary colon cancer spheroids, independent of the mutation status of APC. Indicated cells were lysed and the main components of the destruction complex were co-immunoprecipitated with anti-β-catenin/APC antibody. P1 and P3 show APC truncation, whereas in P2 wild-type APC was detected. Representative examples of three independent experiments are shown. (b) P3 LEF/TCF cells were treated for 72+72 h with indicated amounts of IWP12. Luciferase assay was normalized to viability assessed in parallel using the CellTiterGlo assay. (c) P3 and P1 cells were treated as inband then the CellTiterGlo assay was made. (b,c) Data from five (P3) and four (P1) independent experiments are shown as mean±s.e.m. Figure 8: Wnt secretion is important for the survival of colon TICs. ( a ) Destruction complex is functional in primary colon cancer spheroids, independent of the mutation status of APC. Indicated cells were lysed and the main components of the destruction complex were co-immunoprecipitated with anti-β-catenin/APC antibody. P1 and P3 show APC truncation, whereas in P2 wild-type APC was detected. Representative examples of three independent experiments are shown. ( b ) P3 LEF/TCF cells were treated for 72+72 h with indicated amounts of IWP12. Luciferase assay was normalized to viability assessed in parallel using the CellTiterGlo assay. ( c ) P3 and P1 cells were treated as in b and then the CellTiterGlo assay was made. ( b , c ) Data from five (P3) and four (P1) independent experiments are shown as mean±s.e.m. Full size image We then tested whether truncated APC in colon cancer stem cells is functional as shown above for colon cancer cell lines. Consistently, we found that GSK3β and Axin1 bind to truncated APC and β-catenin in all three spheroid cultures independent of their APC mutation status ( Fig. 8a ). We further tested whether inhibition of Wnt secretion by a Porcupine inhibitor (IWP12) reduced the LEF/TCF–Wnt-reporter signalling in TICs with truncated APC. Similar to colon cancer cell lines, inhibition of Wnts secretion led to a reduction of Wnt signalling and reduces viability of these cells ( Fig. 8b,c ). Taken together, we conclude that high Wnt pathway activation in primary colon cancer cells relies on Wnt secretion, despite mutation in APC, indicating that the level of Wnt signalling is modulated by the secretion of Wnt proteins. In colon cancer, mutations in APC or β-catenin are known to be tightly associated with the transformation of normal epithelia, leading to dysplasia and early adenomas. However, the functional effects of these mutations on the Wnt/β-catenin signalling pathway and the mechanisms whereby they contribute to carcinogenesis are not yet fully understood. Here we provide evidence that sustained Wnt secretion is important for the proliferation and survival of colon cancer cells, both ex vivo and in vivo . Cells carrying mutations in APC or β-catenin are still dependent on the Wnt/β-catenin pathway activation upstream of the β-catenin destruction complex ( Fig. 9 ). Blocking upstream signalling by depleting the Wnt cargo receptor Evi/Wls significantly reduces the proliferation of colon cancer cells. Our results suggest that truncations of the APC tumour suppressor do not render cells independent of exogenous Wnt ligands, but rather lower the threshold of pathway activation by Wnt proteins. 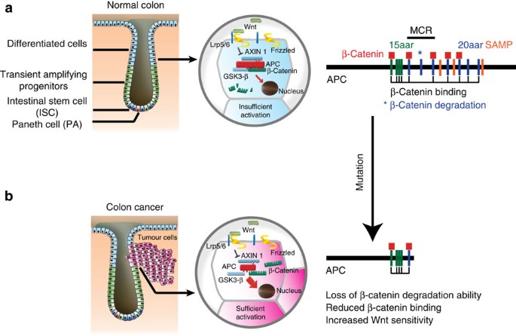Figure 9: Schematic model on the role of Wnt secretion in APC mutant cells. (a) In normal colon cells, Wnt signalling gradients originating at the bottom of colonic crypts determine cell identity. Low amounts of Wnt signalling lead to differentiation of epithelial cells of the colon. Under these conditions, wild-type APC serves as a scaffold, binding β-catenin and catalytic components of the destruction complex, thus sequestering it in the cytoplasm and causing its degradation. (b) In colon cancer cells, APC is truncated but retains some ability to bind β-catenin and act as a scaffold for the destruction complex. However, the efficiency of β-catenin retention is reduced in a manner related to the length of the truncated APC protein. Thus, APC truncations sensitize to canonical Wnts, allowing cancer cells to be more sensitive to activation by Wnt ligands, while retaining regulatory activity throughout the signalling cascade. Further, colon cancer cells acquire the ability to secrete Wnts in an autocrine manner, rendering the tumour increasingly independent of the original Wnt sources of the colonic crypts. Figure 9: Schematic model on the role of Wnt secretion in APC mutant cells. ( a ) In normal colon cells, Wnt signalling gradients originating at the bottom of colonic crypts determine cell identity. Low amounts of Wnt signalling lead to differentiation of epithelial cells of the colon. Under these conditions, wild-type APC serves as a scaffold, binding β-catenin and catalytic components of the destruction complex, thus sequestering it in the cytoplasm and causing its degradation. ( b ) In colon cancer cells, APC is truncated but retains some ability to bind β-catenin and act as a scaffold for the destruction complex. However, the efficiency of β-catenin retention is reduced in a manner related to the length of the truncated APC protein. Thus, APC truncations sensitize to canonical Wnts, allowing cancer cells to be more sensitive to activation by Wnt ligands, while retaining regulatory activity throughout the signalling cascade. Further, colon cancer cells acquire the ability to secrete Wnts in an autocrine manner, rendering the tumour increasingly independent of the original Wnt sources of the colonic crypts. Full size image Our findings are interesting with regards to the observation that extracellular inhibitors of the Wnt/β-catenin signalling, Dkk4 and Sfrps, are frequently downregulated in colorectal cancers [14] , [15] . These proteins had been proposed to have novel functions given the earlier assumption that mutations in APC or β-catenin would render cells completely independent of canonical Wnt/β-catenin signalling. Our results offer a different explanation: as Wnt/β-catenin signalling remains critical for proliferation, reduced expression of secreted Wnt/β-catenin antagonists and high expression of Wnts and Evi/Wls promotes tumourigenesis. The discovery of Evi/Wls as the cargo receptor for all Wnt proteins opened new avenues for addressing whether the production of Wnt ligands is required in cells that harbour APC or β-catenin mutations. Evi/Wls was found to be essential during development, because it is required for the export of all Wnt proteins [9] , [11] . We observed increased expression of Evi/Wls and Wnt ligands in colon cancers, and detected them throughout the whole tissue, as opposed to weak or very localized expression in healthy tissue (for example, Paneth-like cells, lamina muscularis mucosae). This suggests that colon cancer cells are not only dependent on secreted Wnt ligands but also acquire autocrine Wnt secretion capabilities. Notably, upregulation of Wnts or Evi/Wls in colorectal cancer is associated with lower overall survival. Consistently, TCGA recently showed that colon cancer (tissues) display upregulation of Fzd10 and downregulation of DKK1-4 mRNA levels [3] . This, as well as the silencing of SFRPs, supports a model whereby the destruction complex is regulated by upstream signals in colorectal cancers. These results also provide possible explanations for the uneven distribution of nuclear β-catenin [20] , [46] and the clustering of mutations in APC [47] in colon cancer. Mutations in APC most often occur in the mutation cluster region (1,286–1,513 aa), whereas a complete deletion of the APC locus is extremely rare [36] , [39] , [48] , [49] . The retention of truncated APC has alternatively been attributed to its role in cell division [50] , [51] , C-terminal binding protein (CtBP)-dependent oligomerization [52] or to limit excessive levels of β-catenin in the nucleus [53] , [54] . It has also been proposed that certain truncations of APC are selected to ensure that the Wnt/β-catenin signalling pathway is activated to a degree optimal to support tumour growth [37] , [47] . Regulation of β-catenin in colon cancer cells could also be dependent on the APC-like protein, the closest homologue of APC [55] . Our results are consistent with previous studies on overexpressed APC protein fragments of different length, which were shown to retain the β-catenin-binding ability and reduce the signalling activity [40] , [41] , [42] . Importantly, such a model requires that mutant forms of APC remain, at least in part, a functional component of the destruction complex. Accordingly, truncating mutations in APC represent hypomorphic rather than complete loss-of-function alleles, as suggested by Gaspar and Fodde [38] , based on experiments in familial adenomatous polyposis (FAP) mouse models. Genetic studies in mice also demonstrated that APC truncations select for a certain amount of Wnt/β-catenin pathway activation and show a dosage effect in TopFlash reporter assays conducted in mouse ES cells [47] , [56] , [57] . Our study provides further mechanistic evidence that endogenous truncated APC indeed retains the ability to bind β-catenin. Notably, APC proteins have several β-catenin-binding repeats (15 amino-acid repeats (AARs) and 20 AARs), which enable the wild-type form to bind to multiple β-catenin proteins ( Figs 5a and 8 ). Truncated APC proteins that have been associated with colorectal cancer usually retain several of these AAR repeats. Thus, they have the ability to productively engage β-catenin in the destruction complex. Further, we observed that even the shortest APC protein (in Colo320 cells) is able to bind to β-catenin despite a complete lack of known β-catenin-binding repeat regions, indicating that additional interfaces between APC and β-catenin may exist. It has recently been shown that partial silencing of APC can lead to colon cancer in the absence of biallelic mutations in APC [49] . This directly relates to our finding that partial reduction of APC can sensitize RKO cell to Wnt ligands, arguing that mutations in APC create a special situation of reduced β-catenin binding and processing ability. Taken together, these data support a model, whereby colon cancer cells with truncated APC remain susceptible to regulation by upstream signals. Do colon cancers create their own Wnt-dependent niche? High Wnt pathway activity is essential to maintain the stem cell and transient amplifying progenitor compartment in intestinal crypts, and elevated Wnt/β-catenin pathway activity is associated with stem cell signatures in cancer. It is tempting to speculate that colon cancer cells generate a ‘niche’ that enables them to retain an undifferentiated and stem cell-like behaviour, whereas non-cancerous colon stems cells require the crypt microenvironment to provide Wnt and other ‘stemness’ signals [22] . In the case of tumours, the secretion of Wnt ligands and autocrine activation of canonical receptors may have a crucial role in maintaining stem cell populations independent of signals from the microenvironment. Thus, despite the presence of pathway-activating mutations in APC or β-catenin, the survival of colon cancer cells remains dependent on secreted Wnt ligands, and thus requires the activity of the Wnt cargo receptor Evi/Wls. The expression levels of both Wnt3 and Evi/Wls correlate with the degree of colon tumour differentiation, that is, the grade, which in turn correlates with prognosis [24] . The development of small-molecule Wnt antagonists for the treatment of colon cancer has focused on targets downstream of, or at the same level as, the destruction complex. Large-scale sequencing of human colon cancers has revealed recurrent genetic aberrations in a number of signal transducers, including components of the canonical Wnt pathway [58] . In addition, functional screening has uncovered a number of potential targets that act just upstream of the destruction complex. Our results indicate that the pathway can be inhibited further upstream, for example, through inhibitors of Wnt production acting at the level of Porcupine or the Wnt cargo receptor Evi/Wls to regulating Wnt signalling in colon tumours at the site of production. Cell culture All cell lines were obtained from ATCC. HEK293T, MDA-MB231 (DMEM; Gibco), HCT116, HT29 (McCoy’s; Gibco), LoVo, SW480 and DLD1 (RPMI; Gibco) cells were cultured without antibiotics, unless they were stably transfected or transduced. All media were supplemented with 10% fetal bovine serum (PAA). HCT116 TCF4/Wnt cells were cultured in the presence of 50 μg ml −1 hygromycin B, and HCT116 TCF/LEF cells were cultured in the presence of 10 μg ml −1 puromycin. Primary colon cancer-initiating cells Primary human colorectal cancer or derived metastasis were obtained from the University Hospital Heidelberg in accordance with the Declaration of Helsinki. From each patient, informed consent on tissue collection as approved by the University Ethics Review Board was available. Primary human tissue was minced and digested using dispase (BD Biosciences), filtered and cells were seeded in ultralow attachment in cancer stem cell (CSC) media under serum-free conditions with the addition of fibroblast growth factor (FGF) basic (10 ng ml −1 ) and epidermal growth factor (EGF) (20 ng ml −1 ; both from R&D Systems) to allow spheroid formation [45] . For experimental seeding, spheroid cultures derived from three individual patients (P1 (K-Ras, p53 mutant), P2 (p53 mutant) and P3 (K-Ras, PI3CA, p53 mutant)) were dissociated to a single-cell solution by mechanical disruption via pipetting or by accutase treatment. To generate stable LEF/TCF–Wnt-reporter spheroid cultures, P3 spheroids were dissociated, lentivirally transduced using Viromag R/L beads (OZbiosciences) and subsequently cultured in the presence of 5 μg ml −1 puromycin to select for transduced cells. Quantitative PCR Complementary DNA was prepared from 0.5 or 2 μg total RNA, using the RevertAid H Minus First Strand cDNA Synthesis Kit (Thermo Fischer Scientific). Subsequently, the cDNA was diluted to 5 ng μl −1 and used for quantitative PCR on the Lightcycler 480 (Roche), using the universal probe library system (Roche) in a 384-well format. GAPDH and UBC were used as reference genes for relative quantification. Oligos for quantitative PCR are shown in Supplementary Table S1 . Cell-based assays and recombinant proteins siRNAs were obtained from Ambion (Applied Biosystems). Cells were transfected using a total of 0.1% DharmaFECT 1 (Thermo Fischer Scientific) or RNAiMax (Invitrogen). For plasmid transfection, cells were transfected with 10–60 ng DNA (total) per 384-plate well using TransIT reagent (VWR). Cell viability was determined using the CellTiterGlo assay (Promega) according to the manufacturer’s protocol. Recombinant mouse Wnt3a(315-20) was obtained from PeproTech and mouse recombinant R-spondin1 (3474-RS) from R&D Systems. siRNA sequences are shown in Supplementary Table S2 . Full sized scans of all western blots are provided in Supplementary Figure S10 . Generation of stable cell lines To generate stable Evi, control, CTNNB1 knockdown pools or TCF/LEF or LEF–GFP Wnt-luciferase reporter cell lines, we used lentiviral transduction with the indicated constructs. Viral particles were produced using the lentiviral packaging vectors pMDM2-VSVG, psPAX2 and the vector of interest transfected in the ration 3:1:2 into HEK293T cells. Supernatants were collected and filtered (45 μm) 36–42 h post transfection. Two hundred to 500 μl of the supernatant and 2.5 μg ml −1 of polybryne were added to the six-well plate/T125 flask of cells, plate/flask was centrifuged at 2,000 g for 1 h and then incubated for 24–48 h in standard conditions. Stable cell lines were selected in the presence of 20 μg ml −1 puromycin for 72–120 h. Information on sh/shmirRNAs, constructs and antibodies are shown in Supplementary Tables S3–S5 . Mouse xenograft experiments NOD/SCID mice (7–8 weeks, female) were subcutaneously injected with low-passage 3 × 10 5 or 10 × 10 5 (dox experiment) human HCT116 or DLD1 cells lentiviraly transduced with the indicated constructs. shRNA experiments were performed in blinded manner. For induction, shmirEvi/Ctrl mice were treated with 1 mg ml −1 of dox in the drinking water starting from day 18, when the tumour volumes reach around 125–200 mm 3 . Tumour appearance was monitored once or twice per week by palpating the injection area. Experiments were terminated when tumours in control group(s) reached 1,200–1,500 mm 3 . Results for tumour appearance were analysed using R programme and plotted as Kaplan–Meier plot. P -values were counted with the help of the same programme by log-rank test. P -values for difference in tumour volumes was calculated by Student’s t -test. Animal welfare and experimental procedures were performed in accordance with German animal protection law and were approved by the Regierungspräsidium Karlsruhe, Germany (35-9185.81). Immunohistochemistry Immunohistochemical studies were performed on paraffin-embedded slides/sections, and on a Colon-Grade Array with 150 biopsies, including 30 sections each of normal colon, adenoma, and colon cancer grade 1, 2 and 3 tissues. In addition, serial sections from five adenocarcinoma and five normal colon biopsies were analysed. All samples were analysed as approved by the local institutional ethics boards. The samples were kindly provided by the NCT tumour bank for tissue samples. Expression data analysis The data from TCGA ( http://cancergenome.nih.gov/ ) colorectal carcinoma data set (array) was analysed and visualized by Oncomine (Compendia Bioscience, Ann Arbor, MI, USA; http://www.oncomine.org ). Microarray data are preprocessed by Oncomine in a standardized way by log 2 transformation and scaling the median value per microarray to 0. Fold change is calculated as the difference in the means of the normal colon versus adenocarcinoma samples. Cell cycle analysis Cells were seeded 16 h before analysis (20% of confluence), collected and stained with 200 μg ml −1 of propidium iodide, 0.1% sodium azide, 0.1% Triton-X100 and 10 μg ml −1 RNAses for 2–4 h. Single cells were analysed for subG1, S and G2 peaks by fluorescence-activated cell sorting array (BD Bioscience). Analysis was performed with FlowJo. How to cite this article: Voloshanenko, O. et al. Wnt secretion is required to maintain high levels of Wnt activity in colon cancer cells. Nat. Commun. 4:2610 doi: 10.1038/ncomms3610 (2013).